Single-cell and metagenomic analyses indicate a fermentative and saccharolytic lifestyle for members of the OP9 lineage OP9 is a yet-uncultivated bacterial lineage found in geothermal systems, petroleum reservoirs, anaerobic digesters and wastewater treatment facilities. Here we use single-cell and metagenome sequencing to obtain two distinct, nearly complete OP9 genomes, one constructed from single cells sorted from hot spring sediments and the other derived from binned metagenomic contigs from an in situ -enriched cellulolytic, thermophilic community. Phylogenomic analyses support the designation of OP9 as a candidate phylum for which we propose the name ‘Atribacteria’. Although a plurality of predicted proteins is most similar to those from Firmicutes, the presence of key genes suggests a diderm cell envelope. Metabolic reconstruction from the core genome suggests an anaerobic lifestyle based on sugar fermentation by Embden–Meyerhof glycolysis with production of hydrogen, acetate and ethanol. Putative glycohydrolases and an endoglucanase may enable catabolism of (hemi)cellulose in thermal environments. This study lays a foundation for understanding the physiology and ecological role of the ‘Atribacteria’. Over the last ~20 years, cultivation-independent approaches in microbial ecology have dramatically expanded our view of the microbial world [1] , [2] and have revealed that our ability to isolate novel organisms out of the milieu for study remains limited. Although this problem is evident at all taxonomic levels, it is most glaring at the phylum level. Currently, <50% of phylum-level lineages of Bacteria and Archaea have been cultivated and studied in the laboratory [2] , [3] . The vast diversity of these uncultured groups represents an enormous genetic reservoir that has been described as ‘biological dark matter’ to call attention to our profound ignorance of these groups [4] . It can be difficult to discover even the most basic facts about the biology of candidate microbial phyla, because they are often outnumbered in nature. Metagenomics and single-cell genomics are powerful cultivation-independent approaches for probing the nature of so-called ‘dark matter’ organisms by facilitating access to their genomes [5] , [6] . Although metagenomics has allowed the recovery of partial or nearly complete genomes from several candidate phyla in habitats where they are naturally abundant [7] , [8] , [9] , access to less abundant ‘dark matter’ groups has been enhanced by the advent of single-cell genomics, where individual cells are isolated by fluorescence activated cell sorting or micromanipulation techniques including microfluidic sorting, optical trapping and micropipetting; isolated cells are then lysed and the femtogram quantities of DNA released are amplified and sequenced [5] , [6] . Through containment of the sorting and amplification steps within nanoliter reaction volumes, microfluidic approaches ameliorate amplification bias, minimize the amplification of trace DNA contaminants in the sample, laboratory environment and reagents, and allow for detailed observation of cell morphology [10] , [11] , [12] . Complete or partial genomes can be obtained from single cells [10] , [13] , [14] and single-cell genomics has shed light on the possible functions of several candidate phyla [4] , [15] , [16] , [17] , [18] . Here, we take advantage of the complementarity of metagenomics and single-cell genomics to assemble nearly complete genomes of two members of candidate bacterial phylum OP9. Since its discovery in Obsidian Pool in Yellowstone National Park [1] , OP9 has been found in other geothermal springs, petroleum reservoirs, thermal bioreactors and digesters, and wastewater sludge treatment plants [19] , [20] , [21] , [22] , [23] . This distribution demonstrates an affinity for thermal, anaerobic environments, but no genetic data pertaining to OP9 other than PCR-amplified 16S rRNA gene sequences have been reported. We compare single-cell genomic data from 15 OP9 cells isolated from hot spring sediments at Little Hot Creek, CA, (LHC) [19] with a metagenomic data set from an in situ , ~77 °C cellulolytic enrichment in Great Boiling Spring, NV (GBS) [20] to obtain distinct draft genomes of the OP9 population from each environment. Analysis of the shared features of these two genomes offers the first insights into the cell structure and metabolic capabilities of OP9 lineages present in geothermal systems and suggests that they have a role in biomass degradation in these environments. Morphology-based single-cell sorting targeting OP9 Single-cell sorting, lysis and whole-genome amplification using an optical trap and microfluidic device [14] , [17] , as described in Methods, was performed on cells separated from ~80 °C sediments of the hot spring LHC4 ( Supplementary Fig. S1 ), which were previously shown to be dominated by novel Archaea and Bacteria [19] . Initial efforts surveyed the morphological diversity, with the aim of identifying morphologically distinct ‘dark matter’ groups that could be targeted in subsequent sorting efforts. Rod-shaped cells (on average 0.5 μm wide and 4.5 μm long) were identified as members of the candidate phylum OP9. This morphology was distinctive in the sample and was targeted in two subsequent sorting efforts, the second of which resulted in 15 OP9 single-cell genomes (SCGs) out of 21 total SCGs obtained, as assessed by PCR screens. Thus, the morphology-based sorting approach was effective for this lineage and sample, even though it was present at a relatively low abundance (~0.5% of total cells). Half of the OP9 SCGs obtained had 16S rRNA gene fragments identical to the OP9 sequence previously described from LHC4 (LHC4_L1_A09) [19] , although the others differed by 1–2 bases over the ~600 bp sequenced region. This indicated that the sorted OP9 cells all represented a closely related group and that this lineage was a stable member of the microbial community in LHC4 sediments, given that OP9 was recovered from samples collected on three dates spanning ~22 months. Assembly of a composite OP9-SCG After pyrosequencing, filtering and assembly as described in Methods, 15 SCGs with uniform read %G+C content and contig tetranucleotide word frequencies (TNF) were chosen for further sequencing and reassembly ( Supplementary Fig. S2 ). Resulting individual de novo SCG assemblies ranged from 110–872 kb ( Supplementary Table S1 ). The average nucleotide identity (ANI) between overlapping regions of the SCGs ranged from 96.2–99.4% with an average of 98.8% per SCG, greater than the genomic 95% ANI empirically determined to delineate species [24] . A neighbor-joining tree using a distance matrix based on pairwise %ANI did not reveal distinct clusters within the SCGs ( Supplementary Fig. S3 ). Along with high 16S rRNA gene identity (>99.6%), these data indicate that the 15 SCGs represent a single, species-level group within the OP9 lineage. Given the small initial de novo assembly sizes and the relatively low sequencing depth for SCGs [10] (1.5–20x, assuming a 1.5–3.0 Mb genome typical of thermophiles), we determined that it would be difficult to assemble nearly complete SCGs from these data sets individually. However, because the 15 OP9 SCGs represented a single species, we combined the data sets to construct a composite SCG (cSCG) assembly. 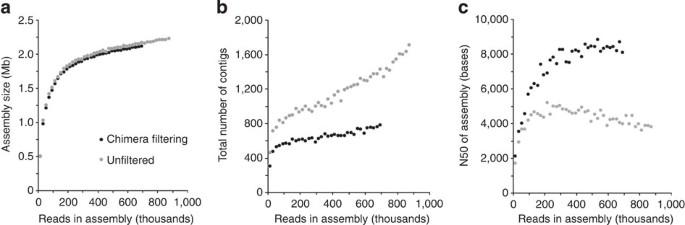Figure 1: Chimera filtering increases contig N50 in the cSCG assembly. Stepwise assembly of composite OP9-SCG before (grey points) or after (black points) filtering out potentially chimeric reads. The increase in (a) total assembly size, (b) number of contigs and (c) contig N50 are shown as a function of the number of reads (resampled at each increment) used. Pooling data from multiple cells alleviates problems inherent in single-cell genomics, such as the random bias in genomic coverage of individual SCGs arising from whole-genome amplification by multiple strand-displacement amplification (MDA) [10] , and resulted in an assembly of ~2.24 Mb ( Table 1 ). Integration of the multiple SCG data sets also enabled application of a jackknifing procedure for removal of chimeric sequences [14] , which occur at a frequency of one chimera per ~10 kb during MDA [10] . This reference-independent chimera-filtering procedure significantly improved the assembly, as evidenced by a >2-fold increase in contig N50 with only a small decrease in overall assembly size despite removal of ~18.5% of total reads ( Fig. 1 , Table 1 ). Table 1 Assembly statistics for the OP9-cSCG and OP9-77CS. Full size table Figure 1: Chimera filtering increases contig N50 in the cSCG assembly. Stepwise assembly of composite OP9-SCG before (grey points) or after (black points) filtering out potentially chimeric reads. The increase in ( a ) total assembly size, ( b ) number of contigs and ( c ) contig N50 are shown as a function of the number of reads (resampled at each increment) used. Full size image Identification of OP9 contigs in a cellulolytic metagenome Principal components analysis of TNF (TNF-PCA) was used to probe metagenomes derived from LHC and another hot spring in the US Great Basin, GBS [18] , located ~400 km north of LHC. Although OP9 reads were present in extremely low abundance in the LHC metagenome, pyrosequencing of 16S rRNA gene fragments amplified from three cellulolytic enrichments incubated at ~77 °C in GBS indicated significant enrichment of OP9 in comparison with undisturbed GBS sediments [25] . TNF-PCA revealed a distinct cluster of contigs from one of these metagenomes (corn stover incubated in spring sediment, ‘77CS’) overlapping with OP9-SCG contigs ( Fig. 2a ), suggesting that this cluster represented genomic fragments from the enriched OP9 lineage, and allowed designation of an OP9 bin (‘OP9-77CS’; Fig. 2a ) of 315 contigs containing ~2.23 Mb. The majority of OP9-77CS contigs displayed a high level of identity to the OP9-cSCG by BLASTN and exhibited a defined read depth within the metagenome (213±50 s.d. ; Fig. 2c ), suggesting a single OP9 phylotype closely related to the OP9-cSCG. Although a portion of OP9-77CS contigs had lower read depth, ~40% of these had >85% identity to the OP9-cSCG, and may be enriched for genes unique to an OP9 strain present at lower abundance in the enrichment. Although some of the contigs in the OP9-77CS bin without BLASTN hits to the cSCG may have originated from organisms other than OP9, they could also represent portions of the OP9 genome that were either not covered or not present in the OP9-cSCG, and were thus retained. 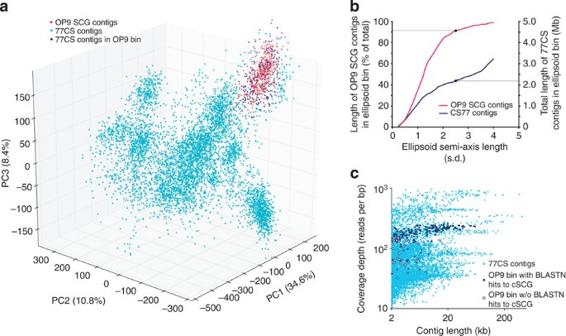Figure 2: Identification of OP9-like contigs from the 77CS metagenome. (a) Principal components analysis (PCA) of tetranucleotide frequency of contigs in the 77CS metagenome and 10 individual OP9-SCG assemblies. The 77CS contigs in dark blue were binned as OP9-like, as defined by their placement within an ellipsoid with a centroid and semi-axis lengths equal to the mean and 2.5 times the s.d., respectively, of the first three principle components (PC1-PC3, with the per cent variation explained by each in parentheses) of the OP9-SCG contigs. Only contigs greater than 2 kb in length are shown. Contigs <2 kb inside this ellipsoid were also included in the OP9 bin if they had significant nucleotide identity (>85% identity over >100 nt) to contigs in the OP9-cSCG by BLASTN. (b) Total length of OP9-SCG and 77CS contigs >2 kb contained within ellipsoids with different semi-axis lengths defined by multiplication of the s.d. of PC1-PC3 of the OP9-SCG contigs by increasing scalar quantities (xaxis). Black points on the curves indicate the multiplier (2.5) used to define the OP9 bin, chosen at an approximate inflection point of the 77CS contig length curve to maximize inclusion of metagenome contigs in the cluster overlapping the OP9-SCGs but minimize inclusion of contigs in adjacent clusters. (c) Plot of coverage depth versus contig length for the 77CS metagenome assembly, highlighting contigs in the OP9 bin with (dark blue circles) and without (open circles) >85% nucleotide identity over >100 bp to the OP9-cSCG assembly. Figure 2: Identification of OP9-like contigs from the 77CS metagenome. ( a ) Principal components analysis (PCA) of tetranucleotide frequency of contigs in the 77CS metagenome and 10 individual OP9-SCG assemblies. The 77CS contigs in dark blue were binned as OP9-like, as defined by their placement within an ellipsoid with a centroid and semi-axis lengths equal to the mean and 2.5 times the s.d., respectively, of the first three principle components (PC1-PC3, with the per cent variation explained by each in parentheses) of the OP9-SCG contigs. Only contigs greater than 2 kb in length are shown. Contigs <2 kb inside this ellipsoid were also included in the OP9 bin if they had significant nucleotide identity (>85% identity over >100 nt) to contigs in the OP9-cSCG by BLASTN. ( b ) Total length of OP9-SCG and 77CS contigs >2 kb contained within ellipsoids with different semi-axis lengths defined by multiplication of the s.d. of PC1-PC3 of the OP9-SCG contigs by increasing scalar quantities ( x axis). Black points on the curves indicate the multiplier (2.5) used to define the OP9 bin, chosen at an approximate inflection point of the 77CS contig length curve to maximize inclusion of metagenome contigs in the cluster overlapping the OP9-SCGs but minimize inclusion of contigs in adjacent clusters. ( c ) Plot of coverage depth versus contig length for the 77CS metagenome assembly, highlighting contigs in the OP9 bin with (dark blue circles) and without (open circles) >85% nucleotide identity over >100 bp to the OP9-cSCG assembly. Full size image Comparison and estimation of completeness of the OP9 genomes The OP9-cSCG and OP9-77CS assemblies displayed a high level of identity and likely represent distinct but closely related species. Each contained full-length 16S rRNA genes that were 98.6% identical. BLASTN revealed reciprocal cSCG-to-77CS coverage of 87.7 and 81.6% with an ANI of 91.9%. These were below the accepted thresholds for 16S rRNA gene identity (98.7%) and genomic ANI (95%) delineating microbial species [3] ; thus, co-assembly of the cSCG and OP9-77CS genomes was not justified. However, the homology and high coverage between the two data sets allowed us to use the OP9-77CS contigs as scaffolds for the cSCG. This scaffolding identified short overlaps among existing contigs and improved the cSCG assembly significantly ( Table 1 ). Because of the high degree of coverage and identity between the two data sets, cross-comparison allowed a rigorous filtering of potential contaminating sequences that could not be accomplished with either data set in isolation. Such filtering, described in Methods, resulted in removal of 9 and 13 contigs from OP9-77CS and OP9-cSCG, respectively, representing ~1% of the assemblies. We have conservatively restricted our prediction of structure and function to genes and pathways present in both the OP9-cSCG and OP9-77CS, representing the core genome from the OP9 lineage present in Great Basin hot springs. Analysis of the predicted protein-encoding genes (coding DNA sequences, CDSs) in the OP9-cSCG and OP9-77CS supported their close relationship and their novelty compared with other genomes ( Table 2 ). One thousand seven hundred sixty CDSs were identified as best-bidirectional hits between the two genomes, with an average predicted protein sequence identity of 94.3%; most CDSs with no BLASTP hit in the other OP9 genome were annotated as hypothetical proteins (73 and 82% for comparison with the 77CS-to-cSCG and cSCG-to-77CS, respectively). The number of CDSs assigned EC numbers by RAST, KAAS and Markov clustering was similar (22.8–35%). The percentages of OP9 CDSs assigned to Clusters of Orthologous Groups (COGs) [26] were 64.6–68%, notably lower than the average of ~80% for genomes of cultivated microbes [27] but comparable with other genomes from previously unsequenced phyla, which are typically enriched with novel CDSs [17] . Table 2 Genomic features of OP9-cSCG and OP9-77CS. Full size table The presence of essential features and highly conserved genes in the OP9-cSCG and OP9-77CS suggested that both data sets represent nearly complete genomes ( Table 2 ). Each contains a complete set of aminoacyl-tRNA synthetases, at least one tRNA gene for each amino acid, and full-length 5S, 16S and 23S rRNA genes. Additionally, all 31 highly conserved genes recognized by AMPHORA [28] were present. An approximate quantification of genome completeness was obtained by comparison with a set of 181 conserved, typically unlinked genes [29] ; the OP9-cSCG and OP9-77CS contained 164 (90.6%) and 167 (92.3%) of these markers, respectively ( Supplementary Table S2 ). However, a majority of the absent markers were genes involved in synthesis of pantothenate and riboflavin, precursors of coenzyme-A (Co-A) and flavin adenine dinucleotide, respectively. The presence of energy-coupling factor transporters specific for these precursors, as well as all necessary genes to subsequently convert them into Co-A and flavin adenine dinucleotide, suggests that the absence of genes for synthesis of pantothenate and riboflavin is due to dependence of OP9 on uptake of these substrates. If these 13 markers are excluded from the analysis, estimated completeness of the cSCG and OP9-77CS are >96% ( Table 2 ), providing a level of confidence for inference of the presence and absence of metabolic capabilities based on gene content. Of the markers detected, only a small minority were present in greater than one copy in each assembly. In approximately half of these cases, the extra markers were present on large contigs and were conserved (>90% identical and in the same genomic context) in both OP9 data sets, suggesting that they are genuinely present in multiple copies. When these are excluded, only 1.8% (3/164) and 4.8% (8/167) of the observed markers were present in greater than one copy. Given that not all of the markers are present in a single copy in all organisms, this analysis suggests a high fidelity for the assemblies, particularly for the OP9-cSCG. Phylogeny and cell envelope structure Phylogenies inferred from 16S rRNA gene sequences ( Fig. 3a ) and 31 conserved protein-coding genes ( Fig. 3b ) support the designation of OP9 as a phylum-level lineage in the Bacteria. OP9 comprises four distinct clades in the 16S rRNA gene-based phylogeny. The OP9-cSCG and OP9-77CS fall within one family-level clade, which inhabits terrestrial geothermal environments world-wide, including the US Great Basin, Yellowstone National Park, China and Kamchatka ( Fig. 3a ; additional OP9 sequences and references in Supplementary Table S3 footnote). Although the OP9 lineage clustered with the JS1 clade with weak bootstrap support, JS1 has been defined as a candidate phylum in its own right by some analyses [30] . Rigorous determination of whether these two clades represent distinct phyla or classes within a single phylum will require analysis of additional phylogenetic markers from JS1, which are currently unavailable. 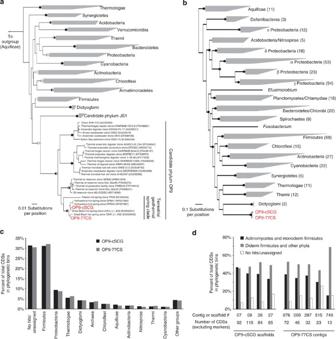Figure 3: Relationship of OP9-SCG and OP9-CS77 to other bacterial groups. (a) Neighbor-joining tree based on a distance matrix of 1,349 aligned positions of 16S rRNA genes from selected bacterial phyla with cultured representatives and the candidate phyla JS1 and OP9, including those in the OP9-SCG and OP9-CS77 assemblies. Black (100%), grey (>80%) and white (>50%) circles indicate bootstrap support (100 pseudoreplicates) for selected nodes in phylogenies inferred using neighbor-joining (left half of circle) and maximum-likelihood (right half) methods. (b) Maximum-likelihood phylogeny inferred from concatenated alignments of predicted amino acid sequences of 31 housekeeping genes identified by AMPHROA in genomes representing a variety of bacterial phyla and the OP9-SCG and OP9-CS77 assemblies. The number of genomes represented in each wedge is indicated in parentheses, and black circles indicate bootstrap support of >80% for 100 pseudoreplicates. (c) Binning of CDSs in the OP9 assemblies based on the phylogenetic affiliation of their top BLASTP hit to a database of sequenced bacterial and archaeal genomes. Phylogenetic groups with fewer than 1% of top hits were aggregated (‘other groups’). (d) Phylogenetic binning of CDSs on contigs or scaffolds containing markers diagnostic for a diderm cell envelope structure31, emphasizing that top BLASTP hits were distributed among both monoderm and diderm Bacteria. Diderm Firmicutes includes members of the Negativicutes and Halanaerobiales. Figure 3: Relationship of OP9-SCG and OP9-CS77 to other bacterial groups. ( a ) Neighbor-joining tree based on a distance matrix of 1,349 aligned positions of 16S rRNA genes from selected bacterial phyla with cultured representatives and the candidate phyla JS1 and OP9, including those in the OP9-SCG and OP9-CS77 assemblies. Black (100%), grey (>80%) and white (>50%) circles indicate bootstrap support (100 pseudoreplicates) for selected nodes in phylogenies inferred using neighbor-joining (left half of circle) and maximum-likelihood (right half) methods. ( b ) Maximum-likelihood phylogeny inferred from concatenated alignments of predicted amino acid sequences of 31 housekeeping genes identified by AMPHROA in genomes representing a variety of bacterial phyla and the OP9-SCG and OP9-CS77 assemblies. The number of genomes represented in each wedge is indicated in parentheses, and black circles indicate bootstrap support of >80% for 100 pseudoreplicates. ( c ) Binning of CDSs in the OP9 assemblies based on the phylogenetic affiliation of their top BLASTP hit to a database of sequenced bacterial and archaeal genomes. Phylogenetic groups with fewer than 1% of top hits were aggregated (‘other groups’). ( d ) Phylogenetic binning of CDSs on contigs or scaffolds containing markers diagnostic for a diderm cell envelope structure [31] , emphasizing that top BLASTP hits were distributed among both monoderm and diderm Bacteria. Diderm Firmicutes includes members of the Negativicutes and Halanaerobiales. Full size image Genome-wide comparison of the OP9-cSCG and OP9-77CS with other Bacteria suggested a relationship with Gram-positive members of the phylum Firmicutes, although key genes indicated that OP9 is diderm (that is, has an outer membrane). A plurality of predicted proteins in the OP9 genomes had top BLASTP hits to members of the Firmicutes, both when all CDSs were considered ( Fig. 3c ) and when CDSs assigned to COGs were first divided into 20 major functional COG categories, ranging from 13 to 244 CDSs for a given category. The majority (>85%) of these top BLASTP hits were to proteins in members of the Firmicutes known or expected to have a monoderm, Gram-positive-like cell envelope structure. However, several genetic markers found exclusively in diderm Bacteria were present in both OP9 genomes, including proteins involved in outer membrane protein assembly (BamA/YaeT, OmpH), secretion across the outer membrane (TolC, TonB, secretin) and the flagellar P- and L-rings (along with other flagellar and chemotaxis genes) associated with the peptidoglycan and outer membrane in diderm Bacteria ( Supplementary Table S4 ) [31] . Top BLASTP hits (average of 48% identity) of CDSs in contigs or scaffolds containing these markers were distributed in both monoderm and diderm taxa ( Fig. 3d ) and were generally similar to the distribution of top BLASTP hits of CDSs throughout the assemblies, suggesting that these markers are genuine parts of the OP9-cSCG and OP9-77CS lineages and not recently obtained by horizontal gene transfer from known diderm taxa. Genes involved in synthesis and export of lipid A ( lpxABCD ; msbA ), a core component of the outer membrane of many diderm Bacteria, were present, but no recognizable homologues of genes required for production and attachment of keto-deoxyoctulosonate and the liposaccharide inner core were found. The OP9 outer membrane structure therefore likely differs from that of other diderm Bacteria containing typical lipopolysaccharide. Potential role of OP9 in (hemi)cellulolysis The presence of CDSs for both extracellular and cytoplasmic glycohydrolases indicate the potential for degradation and utilization of cellulose or hemicellulose by OP9. Both genomes encode an endo-1,4-β-glucanase with a putative N-terminal secretion signal peptide, indicating potential for extracellular activity ( Fig. 4 ). The closest characterized homologues of this gene (31–38% amino acid identity) are an endoglucanase in Pyrococcus furiosus (EglA) [32] and a cellulase in Thermotoga maritima (CelA) [33] , both of which belong to the GH12 family of glycohydrolases [34] . Alignment of the OP9 endo-1,4-β-glucanases with members of GH12 indicate that two glutamates predicted to be involved in catalysis are conserved in the OP9 CDSs (positions 167 and 256). The T. maritima CelA is active on soluble glucans, while the P. furiosus EglA is active on crystalline cellulose and glucan oligosaccharides; both enzymes displayed weak activity on xylan [32] , [33] . Several members of the GH12 family have the capacity for hydrolysis of xyloglucan, a major component of hemicellulose in primary plant cell walls, and it has been suggested that xyloglucanase activity may be an ancestral trait of the GH12 family [35] . Although it is difficult to predict the precise activities of the OP9 endo-1,4-β-glucanase, it is likely involved in hydrolysis of one or more components of (hemi)cellulose. OP9 apparently lacks the capacity for degradation of the lignin component in lignocellulose, as only a single putative dioxygenase (COG1355) and no feruloyl esterases (for example, pfam07519) were observed in the assemblies. 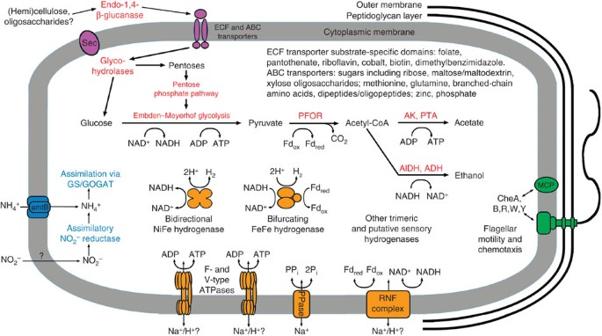Figure 4: Overview of features and potential metabolic capabilities of the OP9 lineage represented by the OP9-SCG and OP9-CS77 genomes as discussed in the text. CDSs in the OP9-cSCG and OP9-77CS associated with predicted functions are listed inSupplementary Table S5. Proteins involved in specific processes are identified by colour: secretion and transporters (purple); saccharide catabolism and fermentation (red); energy conservation (orange); flagellar motility and chemotaxis (green); and nitrogen transport and assimilation (blue). Substrates and products are not necessarily balanced in the reactions depicted. Abbreviations not indicated in the text: ABC, ATP-binding cassette; Fdox, oxidized ferredoxin; AK, acetate kinase; PTA, phosphotransacetylase; AlDH, aldehyde dehydrogenase; ADH, alcohol dehydrogenase; PPi, pyrophosphate; Pi, inorganic phosphate; PFOR, pyruvate-ferredoxin oxidoreductase; PPase, pyrophosphatase; ATPases, ATP synthases; MCP, methyl-accepting chemotaxis protein. Figure 4: Overview of features and potential metabolic capabilities of the OP9 lineage represented by the OP9-SCG and OP9-CS77 genomes as discussed in the text. CDSs in the OP9-cSCG and OP9-77CS associated with predicted functions are listed in Supplementary Table S5 . Proteins involved in specific processes are identified by colour: secretion and transporters (purple); saccharide catabolism and fermentation (red); energy conservation (orange); flagellar motility and chemotaxis (green); and nitrogen transport and assimilation (blue). Substrates and products are not necessarily balanced in the reactions depicted. Abbreviations not indicated in the text: ABC, ATP-binding cassette; Fd ox , oxidized ferredoxin; AK, acetate kinase; PTA, phosphotransacetylase; AlDH, aldehyde dehydrogenase; ADH, alcohol dehydrogenase; PP i , pyrophosphate; P i , inorganic phosphate; PFOR, pyruvate-ferredoxin oxidoreductase; PPase, pyrophosphatase; ATPases, ATP synthases; MCP, methyl-accepting chemotaxis protein. Full size image Several cytoplasmic glycohydrolases encoded in the OP9 genomes could allow for utilization of oligosaccharides derived from cellulose and hemicellulose degradation, including xyloglucan. Both OP9 genomes encode an α-xylanase and β-glucosidase for degradation of isoprimeverose subunits of xyloglucan into glucose and xylose [36] , as well as an α-N-arabinofuranosidase that could act on the L -arabinose-substituted isoprimeverose. The OP9-77CS additionally encodes a β-galactosidase and α- L -fucosidase, which would allow for complete breakdown of all major types of xyloglucan oligomers into hexoses and pentoses. The β-glucosidase would also mediate hydrolysis of cellobiose and longer chain β-glucans. Both genomes additionally encode a β-xylanase, β-mannosidase and amylopullulanase that could facilitate hydrolysis of xylan, mannan and alpha-linked glucan oligosaccharides, respectively. Central metabolism Catabolic capacity of the OP9-cSCG and OP9-77CS appears mainly limited to utilization of hexoses and pentoses via Embden–Meyerhof glycolysis and the pentose phosphate pathway ( Fig. 4 ). The resulting pyruvate could be converted by pyruvate-ferredoxin oxidoreductase to acetyl-coenzyme-A, which could either be processed to acetate with concomitant production of ATP via acetate kinase and phosphoacetyl transferase or be reduced to ethanol by aldehyde and alcohol dehydrogenases. An incomplete tricarboxylic acid cycle and the absence of most genes for NADH:ubiquinone oxidoreductase (Respiratory Complex 1), cytochromes, cytochrome oxidases and quinone synthesis suggests a reliance on fermentation, while the absence of catalase and presence of oxygen-sensitive enzymes such as pyruvate-ferredoxin oxidoreductase indicate an anaerobic lifestyle. Ethanol and acetate, along with carbon dioxide and H 2 (see below) are likely the major fermentation products, as genes involved in production of lactate and butyrate and other common fermentation pathways were not detected. Pathways for catabolism of amino acids and fatty acids are largely absent. Although prediction of the full metabolic capacity is difficult due to the novelty of OP9, these data nonetheless suggest a prominent role for saccharide fermentation and are consistent the enrichment of OP9 on (hemi)cellulose substrates in GBS. The OP9 genomes encode anabolic pathways for most important metabolites, but appear to be dependent on uptake of several vitamins. Neither genome contained evidence for carbon fixation pathways, indicating a heterotrophic lifestyle. Complete or nearly complete biosynthetic pathways for all amino acids except methionine were detected, as well as apparent capacity for de novo synthesis of purines, pyrimidines, NAD(P) and fatty acids. Although OP9 has the capacity for synthesis of pyridoxine, it lacks pathways for synthesis of most other vitamins. The uptake of biotin, folate, pantothenate, riboflavin and dimethylbenzimidazole is likely mediated by energy-coupling factor transporters, as substrate binding domains specific for these vitamins are all present [37] . Ammonia uptake and assimilation appears to be mediated by an Amt transporter and the glutamine synthetase/glutamate-2-oxoglutarate amino transferase pathway, respectively. Two CDSs in the glutamine synthetase/glutamate-2-oxoglutarate amino transferase locus with similarity to assimilatory nitrite reductases may allow utilization of nitrite as an alternative nitrogen source, but no transporters for nitrite were detected. OP9 appears to be dependent on sulphide as a sulphur source because genes encoding assimilatory sulphate reductase were not present. Energy conservation In addition to ethanol production, regeneration of oxidized electron carriers could be mediated by several cytoplasmic hydrogenases, including one NiFe hydrogenase and four FeFe hydrogenases ( Fig. 4 ). The large subunit of the tetrameric NiFe hydrogenase clusters with group 3b bifunctional hydrogenases ( Supplementary Fig. S4 ) [38] , which includes sulfhydrogenases of thermophilic Archaea that can catalyse reduction of sulphur to sulphide in addition to hydrogen production [39] . Two of the FeFe hydrogenases cluster with group A1 and A8 trimeric NAD(P)-linked hydrogenases ( Supplementary Fig. S5 ) [40] . The subunits of one of these shares 44–56% identity to those of a recently described ‘bifurcating’ hydrogenase in Thermotoga maritima , which couples H 2 production to concomitant oxidation of NADH and reduced ferredoxin (Fd red ) [41] and may allow for proton reduction at relatively high H 2 concentrations. The remaining two FeFe hydrogenases cluster with groups C and D, which are poorly characterized but may have a regulatory role due to the presence of PAS domains (Group C) and their association with protein kinases and phosphatases [40] . Maintenance of a chemiosmotic membrane potential appears to be mediated primarily by an RNF complex, a membrane-associated pyrophosphatase, and two ATP synthases. RNF is a membrane-bound, six-subunit complex capable of energy conservation by coupling ferredoxin:NAD + oxidoreductase activity with H + or Na + transport [42] . Depending on the intracellular redox state (balance of NADH and Fd red ), the RNF complex could either allow production of a membrane potential by oxidation of NAD + with Fd red , or production of Fd red from NADH by reverse electron transport. Accordingly, two ATP synthases (F-type and V-type) could allow for either ATP production from a chemiosmotic membrane gradient generated by the RNF complex or generation of membrane potential by ATP hydrolysis. The pyrophosphatase and F-type ATP synthase appear to mediate Na + and H + transport, respectively, based on several conserved residues ( Supplementary Fig. S6 ) [43] , [44] , suggesting that both Na + and H + are involved in maintenance of membrane potential. The OP9-cSCG and OP9-77CS genomes described here offer the first significant insights into the metabolic capabilities and ecology of this ‘dark matter’ group. Our analyses of the core genome of hot spring OP9 lineages, which focus on basic cell structure and central metabolism, indicate an anaerobic, fermentative, saccharolytic lifestyle with the potential for degradation of (hemi)cellulose. This is consistent with the observed enrichment of OP9 on cellulosic biomass incubated in the hot spring GBS [25] and supports the hypothesis that OP9 is actively involved in biomass degradation in thermophilic, cellulolytic microbial consortia. It is tempting to extend this prediction to other members of the OP9 lineage, which tend to be found in thermal, anaerobic environments with large amounts of biomass. The potential for utilization of xyloglucan may carve out a niche for OP9, and could explain its low-level but consistent presence in these environments. The apparent reliance of OP9 on exogenous vitamins suggests a dependence on other organisms in the in situ enrichments, corroborated by the presence of COGs involved in de novo vitamin synthesis elsewhere in the 77CS metagenome. These results facilitate enrichment strategies targeted at cultivation of OP9 and pave the way to understanding the role of this candidate phylum. This study also illustrates the utility of combining single-cell and metagenomics approaches, even in cases where data sets originate in distinct species or environments. Based on data presented here, we propose the taxonomic epithets ‘ Candidatus Caldatribacterium californiense’ and ‘ Ca. Caldatribacterium saccharofermentans’ to refer to the OP9-cSCG and OP9-77CS phylotypes, respectively. The descriptions of the taxa are as follows: ‘Caldatribacterium’ (Cald.atri.bac.te'ri.um. L. adj. caldus, hot; L. adj. ater -tra -trum, black; L. neut. n. bacterium, rod or staff. N.L. neut. n. Caldatribacterium refers to a rod-shaped bacterium from a hot environment, where ‘black’ or ‘dark’ references both microbial ‘dark matter’ and the dark, anaerobic environments where the lineage is found), ‘saccharofermentans’ (sac.cha.ro. fer’men.tans. Gr. n. sakchâr, sugar; L. v. fermento, to ferment; N.L. part. adj. saccharofermentans, sugar-fermenting), and ‘californiense’ (ca.li.for.ni.en’se. N.L. neut. adj. californiense, of or belonging to California). 16S rRNA gene phylogenetics firmly places ‘ Ca. Caldatribacterium saccharofermentans’ and ‘ Ca. Caldatribacterium californiense’ within candidate bacterial phylum OP9 along with 16S rRNA gene phylotypes recovered from a variety of environments, including geothermal systems, petroleum reservoirs, anaerobic digesters and wastewater treatment facilities. In addition, phylogenetic analyses support the proposal for the candidate phylum ‘ Atribacteria ’ (A.tri.bac.te’ri.a. N.L. n. Atribacteria, the ‘dark’ bacterial phylum) inclusive of members of the OP9 lineage. Single-cell sorting, whole-genome amplification, and sequencing An overview of methods used for a combined single-cell genomic and metagenomic analysis targeting OP9 is shown in Supplementary Fig. S1 . Samples for single-cell sorting were prepared from source pool sediment from LHC4 in the Long Valley Caldera, CA, USA [19] . Cells were separated from sediment by centrifugation over a Nycodenz density cushion [45] , stored either on ice/4 °C in ethanol (10%, volume/volume) or on dry ice/−80 °C in betaine (6%, weight/volume), and sorted within 1 week of collection. Measurements of temperature, pH and conductivity of spring water at the collection site were performed using hand-held metres that were calibrated in the field before sampling (LaMotte 5 Series, Chestertown, MD or YSI Model 30, Yellow Springs, OH and WTW Model pH330i, Weilheim, Germany) as described previously [18] , [19] . Single-cell sorting was performed on three separate weeks in October 2009, April 2010 and August 2011 using a microfluidic device mounted on a phase-contrast microscope equipped with a 1 W, 976 nm laser for optical trapping as previously described [17] , except that an updated but functionally analogous microfluidic device with 48 sorting chambers was used. Briefly, the cell sorting system involves loading a mixture of cells into each of two central channels, using the laser to transfer individual cells through gated channels into each of the 48 chambers, lysing them, and amplifying their genomes using MDA. Before loading into the microfluidic device, cells were diluted to ~10 4 cells per μl in PPT buffer (phosphate-buffered saline pH 7.4 with 0.01% pluronic F127 and 0.01% Tween-20) containing 0.1 mg ml −1 BSA (New England Biolabs, Ipswich, MA). In some cases, cells were pretreated with 0.5 μg ml −1 proteinase K to weaken proteinaceous cell envelopes and potentially enhance on-chip lysis [46] ; this pretreatment did not apparently have a significant impact on lysis of cells containing OP9 16S rRNA genes. Additionally, cell samples sorted in April 2010 were mixed with 10 4 copies per μl of a traceable plasmid (pBK-CMV; Agilent Technologies, La Jolla, CA) to control for the presence of extracellular DNA. Cell lysis and whole-genome amplification by MDA were performed in the microfluidic device as described [17] . MDA product subsamples (0.5 μl) were used as template in PCR to amplify either bacterial (primers 9bF and 1512uR) or archaeal (primers 8aF and 1406uR) 16S rRNA genes [19] . PCR products were sequenced from the forward primer using the Sanger method (Functional Biosciences, Madison, WI, USA) and compared with the NCBI non-redundant nucleotide (nr-nt) database using BLASTN [47] . Amplification products from April 2010 were additionally screened for the presence of the traceable plasmid containing a CMV promoter using primers 5′-CATATATGGAGTTCCGCGTTAC-3′, 5′-CGTACTTGGCATATGATACACTTG-3′ and a hydrolysis probe BHQ1-5′-CTGGCTGACCGCCCAACGA-3′-HEX (vector reads were not detected in the MDA product mixtures from cells). Amplified SCGs belonging to the OP9 lineage were further amplified by a second round of amplification, and library preparation and shotgun sequencing was carried out as previously described [17] using custom bar-coded adaptor oligonucleotides to enable pooling of multiple libraries and the 454 FLX platform with Titanium chemistry (Roche, Branford, CT) or alternatively, using the Nextera 454 titanium kit (Epicentre, Madison, WI). In all cases, purified libraries were quantified by digital PCR and normalized before sequencing [48] . Assembly and co-assembly of SCG All pyrosequence reads from SCG libraries were initially filtered for quality using mothur [49] and reads corresponding to trace contamination with human DNA were identified by BLASTN [47] against the human genome database ( ftp://ftp.ncbi.nlm.nih.gov/blast/db/ ) and removed. Assembly of pyrosequence reads from individual SCGs was performed with the ‘Newbler’ GS De Novo Assembler v2.6 (Roche), using default parameters with an expected coverage of 500 and the -urt option. FastQC ( http://www.bioinformatics.babraham.ac.uk/projects/fastqc/ ) was used to examine the %G+C distribution of reads, and the JCVI Multi-Dimensional Scatter Plot Viewer ( http://gos.jcvi.org/openAccess/scatterPlotViewer.html ) [50] was used for TNF-PCA in assembled contigs. A subset of 10 SCGs with nearly identical %G+C read distributions and single, homogenous clustering of contigs by TNF-PCA, thus likely largely free of contamination, were selected. Contigs from these 10 SCGs were used to identify potential contaminants in four other SCGs using hierarchical average correlation clustering of TNF-PCA, with contigs cut into 2 kb fragments with 1 kb overlap. Reads mapping to contigs with one or more fragment falling outside the cluster overlapping with the 10 SCGs were removed, and filtered data sets were reassembled. Per cent ANI of these 14 SCGs plus an additional OP9-SCG were determined by pairwise BLASTN. The resulting distances (100%—%ANI) were used to construct a neighbor-joining tree using Phylip [51] . After further 454 sequencing on a subset of the 15 SCGs chosen for analysis, reads from these SCGs were pooled and a cSCG assembly was made using Newbler. Additionally, a jackknifing procedure was used to remove chimeric reads from the cSCGs [14] . Metagenome sequencing and assembly Cellulosic biomass was incubated at various locations in the hot spring GBS, near Gerlach, NV, USA [18] . A full description of the cellulolytic enrichments is described in Peacock et al . [25] ; methods pertaining to the metagenome used in this study are described below. Twenty grams of ammonia fibre explosion (AFEX)-treated corn stover (CS) sealed in a 100-μm mesh nylon filter bag was incubated buried ~1 cm in the sediment near the outflow of GBS for 64 days. As the average water temperature was 77 °C at the site of incubation of the CS, this sample was designated ‘77CS’. After incubation, the 77CS substrate was harvested, frozen immediately on dry ice and stored at −80 °C. DNA was extracted using the FastDNA Spin Kit for Soil (MP Biomedicals, Solon, OH), ethanol precipitated, and resuspended in TE buffer (10 mM Tris pH 8, 1 mM EDTA). Rapid 454 and standard Illumina libraries were prepared from purified DNA according to manufacturer’s protocols and sequenced on the 454 FLX platform (Roche) using Titanium chemistry and the Illumina GAIIx platform (Illumina, San Diego, CA) using paired-end 150 cycle reads, respectively. This produced a total of 179 Mb of 454 sequence and 13.1 Gb of Illumina data, which were co-assembled using a tiered assembly methodology. In brief, after trimming and quality filtering, the 454 and Illumina reads were initially assembled with Newbler and SOAPdenovo ( http://soap.genomics.org.cn/soapdenovo.html ), respectively. Contigs from the Newbler assembly and multiple SOAPdenovo assemblies using different k-mer lengths were dereplicated and merged using Newbler (contigs <2 kb and remaining unassembled reads) followed by merging of all contigs with Minimus2 [52] . Thresholds for merging contigs were limited to overlaps of 60 bases or greater with >98% identity of the overlap. Validation of the assembly and estimation of contig coverage were performed using read mapping with Burrows-Wheeler Aligner and analysed using Samtools [53] . Metagenome binning and scaffolding of the composite SCG TNF-PCA of the 77CS assembly with the same subset of 10 OP9-SCG contigs described above was performed. 77CS contigs falling within an ellipsoid with a centroid and semi-axis lengths defined by the mean and s.d. of the first three principal components of the OP9-SCG contigs were binned as OP9-like, with the added constraint that 77CS contigs <2 kb were required to have a region of homology (>85% identity over >100 nucleotides) with the OP9-cSCG assembly. This subset of the metagenome, referred to as OP9-77CS, was compared with the OP9-cSCG by BLASTN to determine the reciprocal coverage and per cent ANI. Further assembly and scaffolding of the cSCG contigs was performed manually using the output of the BLASTN analysis. In cases where cSCG contigs overlapped by comparison with the OP9-77CS contigs, the contigs were joined, using the region of the cSCG contig with a higher overall quality score in the region of overlap. SCGs and metagenome analysis The OP9-cSCG and OP9-77CS contigs were submitted to RAST [54] for gene calling and annotation. OP9-cSCG and OP9-77CS data sets were further filtered by BLASTP of predicted CDSs from one OP9 genome into a database containing the other OP9 genome, the RefSeq protein database (Release 52), and a recently sequenced Thiovulum SCG [14] . Contigs where no CDSs had top BLASTP hits to the other OP9 genome, and where at least one CDS had a BLASTP hit with >70% identity to the RefSeq database or the Thiovulum genome, were removed. A single contig in the OP9-77CS containing a portion of a 23S rRNA gene with 98% identity to that of Thermodesulfobacterium sp. OPB45 was also removed; only 10 CDSs on 9 contigs in the OP9-77CS assembly had top BLASTP hits to Thermodesulfobacteria, all of which contained CDSs with top BLASTP hits to OP9-cSCG or other Bacteria, suggesting minimal contamination from this group in the OP9-77CS. Additional annotation of coding sequences predicted by RAST was performed using the KEGG Automatic Annotation Server (KAAS) [55] using a BLAST bit score cutoff of 60, the Conserved Domain Database (CDD) [56] with an e -value cutoff of 1e −5 , and by comparison with a database of proteins assigned to Enzyme Commission (EC) numbers by Markov clustering using BLASTP with a 1e −20 cutoff [57] . A set of single-copy genes conserved in Bacteria were detected and aligned using AMPHORA [28] , and phylogenies were inferred by maximum likelihood using RAxML V. 7.2.6 (ref. 58 ). 16S rRNA genes from OP9 and other Bacteria were initially aligned using the Greengenes NAST server [59] . Distance matrices, bootstrapping and maximum likelihood and neighbor-joining methods were performed using PHYLIP V. 3.6.9 (ref. 51 ). A list of species and accession numbers of sequences used for phylogenetic analyses are shown in Supplementary Table S3 . CDSs from OP9-cSCG and OP9-CS77 were analysed by BLASTP against RefSeq protein database and the results were used to infer the phylogeny of the hits using CHNOSZ V. 0.9-7 (ref. 60 ). Accession numbers: 16S rRNA gene sequences of individual OP9 SCGs (Accession numbers KC110876 to KC110890) have been deposited in GenBank. Nearly complete OP9 assemblies have been deposited as Whole-Genome Shotgun projects at DDBJ/EMBL/GenBank under the accession numbers APCU00000000 (OP9-77CS) and APKF00000000 (OP9-cSCG). The versions described in this paper are the first versions, APCU01000000 (OP9-77CS) and APKF01000000 (OP9-cSCG). Chimera-filtered 454 reads used in the cSCG assembly have been deposited in the Short Read Archive (SRR609896). Annotated assemblies and predicted proteins for the OP9-cSCG (Genome ID 6666666.23228) and OP9-77CS (ID 6666666.23137) are available on the RAST guest account ( http://rast.nmpdr.org , using login and password ‘guest’). Complete 77CS metagenome data are also available in the Integrated Microbial Genomes with Microbiome Samples (IMG/M, http://img.jgi.doe.gov/m ) database, taxon object ID 3300000106. How to cite this article: Dodsworth J. A. et al . Single-cell and metagenomic analyses indicate a fermentative and saccharolytic lifestyle for members of the OP9 lineage. Nat. Commun. 4:1854 doi: 10.1038/ncomms2884 (2013).